The crystallization water of gypsum rocks is a relevant water source for plants Some minerals, like gypsum, hold water in their crystalline structure. Although still unexplored, the use of such crystallization water by organisms would point to a completely new water source for life, critical under dry conditions. Here we use the fact that the isotopic composition of free water differs from gypsum crystallization water to show that plants can use crystallization water from the gypsum structure. The composition of the xylem sap of gypsum plants during summer shows closer values to gypsum crystallization water than to free soil water. Crystallization water represents a significant water source for organisms growing on gypsum, especially during summer, when it accounts for 70–90% of the water used by shallow-rooted plants. Given the widespread occurrence of gypsum in dry lands throughout the Earth and in Mars, these results may have important implications for arid land reclamation and exobiology. Gypsum (CaSO 4 ·2H 2 O) is a rock-forming mineral that also occurs in soil [1] . Gypsum outcrops are widespread throughout the Earth, being present in the five continents [2] . They are particularly prevalent in arid and semi-arid regions of Africa, Western and Central Asia [3] , where they affect ca. 40%, 75% and 25% of the total surface, respectively [4] . Gypsum is also a key water-holding mineral of Mars [5] . Under natural conditions and depending on the temperature, pressure and dissolved electrolytes or organics, gypsum may lose crystallization water molecules, becoming bassanite (that is, hemihydrate: CaSO 4 ·½H 2 O) or anhydrite (CaSO 4 ) [6] , [7] . As crystallization water can account for up to 20.8% of gypsum weight [8] , it has been suggested that it could constitute a relevant source of water for organisms, particularly during summer [4] , [9] . This suggestion is consistent with the phenology observed in some shallow-rooted plants growing on gypsum, which remain active when drought is intense [4] , and with the increased soil moisture of gypsum soils during summer as compared with surrounding non-gypsum soils [10] . However, the possibility that organisms could use crystallization water from gypsum or any other mineral remains unexplored. To assess this hypothesis, we analyze the hydrogen ( δ 2 H) and oxygen ( δ 18 O) isotope composition of the xylem water of the gypsum-specialist plant Helianthemum squamatum (L.) Pers. This species has shallow roots [11] that do not reach the water table [12] , and remains phenologically active during summer [13] . Consequently, the main sources of water available to this and other shallow-rooted plants growing on gypsum hills are free soil water and potentially also gypsum crystallization water. We compare the isotope composition of the xylem sap of plants with that of free and crystallization water of gypsum soils, both in spring and summer. In addition to absolute values, we consider the slope of the δ 18 O/ δ 2 H relationship and the deuterium excess, that is, the deviation from the Global Meteoric Water Line, which describes the typical δ 18 O/ δ 2 H relationship for precipitation [14] . The isotopic composition of the xylem sap of H. squamatum plants is closer to gypsum crystallization water than to free soil water, particularly during summer. The analysis through Bayesian stable isotope mixing models indicates that gypsum crystallization water accounts for up to 90% of the water used by this species during summer. The isotopic composition of H. squamatum plants is similar to that of other plants coexisting in the same community, indicating that the use of crystallization water is a common mechanism to shallow-rooted plants growing on gypsum. These results provide the first experimental evidence in support of the role of gypsum crystallization water as a water source for life. 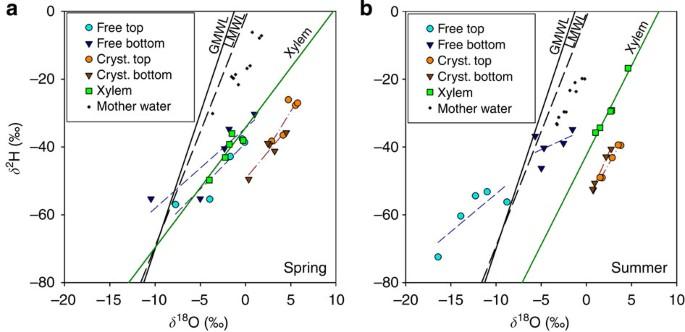Figure 1:δ2H andδ18O composition of the xylem sap ofH. squamatumand the four different sources of water analyzed from gypsum soils. (a) Spring data, (b) Summer data. Global Meteoric water line (GMWL, black continuous) and local meteoric water line in Zaragoza (LMWL, years 2000–2006, black broken) are shown along with lines for the xylem sap of plants (green squares), free soil water from 0–10 cm (light blue dots) and 10–20 cm (dark blue triangles) soil depth, and gypsum crystallization water at 0–10 cm (orange dots) and 10–20 cm (brown triangles). Calculated values of mother water are represented as cross-hairs. Isotopic composition of soil and plant water Free and crystallization water of gypsum soils had different isotopic compositions that varied seasonally ( Supplementary Table 1 ). Free water extracted from the top 10 cm of the soil was less 18 O and 2 H-enriched during summer than in spring, while the opposite change was found in free water extracted from 10–20 cm ( Fig. 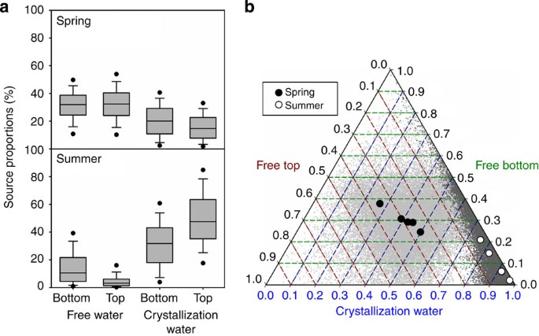Figure 2: Results of Bayesian stable isotope mixing models on the contribution of different sources of water to the xylem sap ofH. squamatumplants. (a) Box plots considering the whole population (two groups, spring and summer,N=5) and four sources (free and crystallization water at two depths). Estimations were calculated from 10,000 posterior iterations per group. (b) Ternary plot showing the results obtained by modelling individual plants (that is, ‘solo’ model). Total contribution of crystallization stands for the sum of crystallization water from the two soil depths analyzed. Circles indicate the average value for each individual (black: spring, white: summer). Dots in the background represent 10,000 posterior iterations per plant (Light grey: spring, dark grey: summer). 1 , Supplementary Table 2 ). The observed enrichment in deeper soil layers is consistent with water undergoing successive evaporative processes from spring to summer [15] , [16] . The remarkably low δ 18 O and δ 2 H of free top soil water during summer is similar to values typically found in the upper layers of very dry soils, and is due to the diffusion of depleted water vapour released from underlying soil layers [15] . Thus, our results indicate that the evaporation front was located within the top 10 cm in spring and within 10–20 cm in summer. Compared with free water, crystallization water had higher δ 18 O, but similar δ 2 H ( Fig. 1 , Supplementary Table 2 ), leading to very low deuterium excess, as reported for other gypsum soils [17] , [18] . This is due to the opposite fractionation factors affecting 18 O and 2 H during gypsum crystallization [17] . Applying these fractionation factors (see Methods), we could estimate values of gypsum mother water that were close to the Local Meteoric Water Line ( Fig. 1 ). The isotopic composition of gypsum crystallization water was homogeneous across soil depths in spring ( Supplementary Table 2 ). However, crystallization water from soil collected at 10–20 cm was more 18 O and 2 H-depleted than that from the top 10 cm of the soil during summer ( Supplementary Table 2 ). Figure 1: δ 2 H and δ 18 O composition of the xylem sap of H. squamatum and the four different sources of water analyzed from gypsum soils. ( a ) Spring data, ( b ) Summer data. Global Meteoric water line (GMWL, black continuous) and local meteoric water line in Zaragoza (LMWL, years 2000–2006, black broken) are shown along with lines for the xylem sap of plants (green squares), free soil water from 0–10 cm (light blue dots) and 10–20 cm (dark blue triangles) soil depth, and gypsum crystallization water at 0–10 cm (orange dots) and 10–20 cm (brown triangles). Calculated values of mother water are represented as cross-hairs. 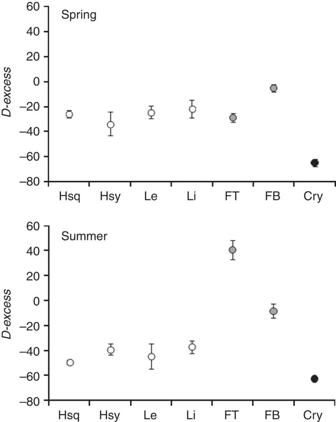Figure 3: Isotopic composition of the xylem sap ofH. squamatumand other coexisting shallow-rooted sub-shrub species and the free and crystallization gypsum water in spring and summer. Plants, free soil water and crystallization water are represented by white, grey and black circles, respectively. Cry, crystallization gypsum water; FB, Free water from the 10–20 cm of the soil; FT, Free water from the top 10 cm of the soil; Hsq,H. squamatum; Hsy,H. syriacum; Le,L. subulatum; Li,L. suffruticosum. Data are presented as mean±s.e.m. Differences among species were not significant after GLM models with ‘species’ and ‘season’ as fixed factors (degrees of freedom=3,F=1.0,P=0.385,N=5). Full size image The isotope composition of the xylem sap of H. squamatum plants also varied between spring and summer ( Supplementary Table 3 ), showing higher δ 18 O and δ 2 H in summer ( Fig. 1 ). The analysis of the most likely sources of water used by H. squamatum plants in spring and summer through Bayesian stable isotope mixing models confirmed that plants used different water sources throughout the year ( Fig. 2 ). In spring, the composition of xylem water was best explained by a combination of free water from the two different depths of the soil analyzed and gypsum crystallization water in balanced proportions ( Fig. 2 ). However, the estimated contribution of water sources changed dramatically in summer, when the total contribution of gypsum crystallization water (that is, the sum of estimated contributions of top and soil crystallization water) accounted for 70–90% of the water in the xylem sap of plants, while the contribution of top free soil water decreased to 0–10% ( Fig. 2 ). Estimated contributions were consistent, regardless of models being determined at the population level (two groups, N =5; Fig. 2a ) or separately for each individual (‘solo’ model, Fig. 2b ). The diagnostic correlation matrix between estimated proportions for each source indicated that the models strongly differentiated free and crystallization water ( Supplementary Fig. 1 ). Figure 2: Results of Bayesian stable isotope mixing models on the contribution of different sources of water to the xylem sap of H. squamatum plants. ( a ) Box plots considering the whole population (two groups, spring and summer, N =5) and four sources (free and crystallization water at two depths). Estimations were calculated from 10,000 posterior iterations per group. ( b ) Ternary plot showing the results obtained by modelling individual plants (that is, ‘solo’ model). Total contribution of crystallization stands for the sum of crystallization water from the two soil depths analyzed. Circles indicate the average value for each individual (black: spring, white: summer). Dots in the background represent 10,000 posterior iterations per plant (Light grey: spring, dark grey: summer). Full size image Drought experiment In-plant fractionation processes could also affect the observed values in xylem water [19] , [20] , [21] . Among them, the most critical under our experimental conditions is the potential evaporative enrichment of xylem water, associated to limited transpiration rates [19] , [21] . To evaluate the residence time of xylem water in H. squamatum , we ran a drought experiment with potted plants. One week of drought (which reduced volumetric water content from 27.6 to 3.7%, Supplementary Fig. 2 ) significantly decreased transpiration, total leaf conductance and internal CO 2 concentrations ( Table 1 , Supplementary Table 4 ). Nevertheless, transpiration rates were maintained over 2 mmol m −2 s −1 and estimated mean residence time of water was ca. 2 h in water-stressed plants ( Table 1 ). All data are available in the Supplementary Data 1–3 . Table 1 Gas exchange measurements of H. squamatum plants included in the control and drought treatments of the pot experiment. Full size table Altogether, our results indicate that H. squamatum uses gypsum crystallization water as a water source, particularly during summer drought. We have strong evidence to discard alternative explanations to the observed isotopic composition of the xylem sap of H. squamatum . First, the different fractionation processes described between soil and xylem water do not match with our observations. Isotope fractionation during water uptake has been described for certain xerophytic plants, but only for 2 H, and in the opposite direction as in our study, that is, water becomes 2 H-depleted [19] . Similarly, it has been suggested that water uptake mediated by mycorrhyza may cause an additional fractionation, based on water extracted from sporocarps of ectomycorrhyzal fungi, but the effect was considered to be negligible (<0.5‰ for δ 18 O) [22] . Fractionation is likely to be even smaller in water transported through mycorrhizal hyphae only (that is, not including sporocarps), since most of such transport is apoplastic, without mixing with the cytoplasm [23] . Second, xylem water could also become progressively 18 O and 2 H-enriched through bark evaporation. However, this is mainly associated with young stems exposed to high evaporative demand, together with long residence times for xylem water [19] , [20] , [21] . This was not our case, since we sampled at the base of the stem, which had a thick and strongly hydrophobic bark, and our pot experiment showed short water residence times under drought (about 2 h for the whole plant). Furthermore, due to differential fractionation factors of 18 O and 2 H (ref. 14 ), if evaporation took place in the xylem, we would expect lower slopes for the δ 18 O/ δ 2 H relationship than in the soil, particularly in summer. In our study, the slope of the δ 18 O/ δ 2 H relationship in xylem water was similar to that of free water in spring ( Fig. 1a ), but was clearly steeper in summer, becoming parallel to both crystallization water and the meteoric water line ( Fig. 1b ). Third, it can be argued that the low deuterium excess of xylem water during summer corresponds to a highly-enriched pool of free water, typical of the evaporation front of dry soils [15] . Although the contrasting isotopic composition of free water from bottom and top soil layers places the evaporation front within the 10–20 cm of the soil, the maximum enrichment of the liquid water at the evaporation front could be higher than measured values at this depth. This could be due to partial contribution of the (depleted) vapour phase to distilled water, or a slightly deeper evaporation maximum, not included within sampling depths, but still available to shallow-rooted plants. However, if plants were only using water from that hypothetical evaporation front, the values in the xylem should be aligned with the gentle slope of the evaporation line of free soil water in the δ 18 O/ δ 2 H bi-plot ( Fig. 1b ). As mentioned before, this was the case in spring, when plants were relying on free water ( Fig. 1a ), but not in summer, when the slope of the line was steeper, and parallel to the meteoric water line ( Fig. 1b ). Overall, these results reinforce our interpretation of the use of gypsum crystallization water, a highly fractionated but non-evaporated water source, by H. squamatum plants during summer. The use of gypsum crystallization water during dry periods seems to be a common feature in shallow-rooted plants growing in the area (including plants not exclusive to gypsum), which showed a similar isotopic composition to H. squamatum during summer ( Fig. 3 ). Our results may further be extrapolated to other organisms growing on gypseous soils with a known ability to dissolve gypsum [24] , hence releasing the water molecules held in its crystalline structure. How do plants manage to obtain crystallization water molecules from gypsum? We suggest two complementary mechanisms: passive uptake through soil heating and active extraction through changes in soil chemistry. Experiments undertaken at atmospheric pressure indicate that the conversion of gypsum to anhydrite is initiated at 42–60 °C (ref. 6 ). However, this temperature threshold may be lower in non-pure gypsum, as the activation energy for the dehydration of gypsum is lower in soils than in pure mineral [25] . Temperatures of the top centimetres of gypsum soils frequently exceed 40 °C during summer [9] , with values of 51 °C being reported at 3-cm depth in some regions [26] , [27] . Under such circumstances, gypsum from the most superficial layers of the soil can be easily dehydrated [28] , releasing water molecules profitable to plants and potentially also other organisms. This may further explain the apparently higher contribution of crystallization water from the top than the bottom soil ( Fig. 2a ). The resulting anhydrite is highly unstable and rehydrates to bassanite in only a few minutes when exposed to air [7] . Such bassanite may dehydrate faster and at lower temperatures than gypsum, rendering unstable anhydrite that is subsequently hydrated, giving rise to successive dehydration—rehydration cycles [7] . Gypsum rehydration may take place overnight, when temperatures cool down, decreasing the vapour pressure of water. This would constitute a water storing system in the soil, periodically recharged by atmospheric moisture without the need of reaching the dew point. Figure 3: Isotopic composition of the xylem sap of H. squamatum and other coexisting shallow-rooted sub-shrub species and the free and crystallization gypsum water in spring and summer. Plants, free soil water and crystallization water are represented by white, grey and black circles, respectively. Cry, crystallization gypsum water; FB, Free water from the 10–20 cm of the soil; FT, Free water from the top 10 cm of the soil; Hsq, H. squamatum ; Hsy, H. syriacum ; Le, L. subulatum ; Li, L. suffruticosum . Data are presented as mean±s.e.m. Differences among species were not significant after GLM models with ‘species’ and ‘season’ as fixed factors (degrees of freedom=3, F =1.0, P =0.385, N =5). Full size image The thermodynamic equilibrium between the different phases of calcium sulphate is also affected by the presence of dissolved electrolytes and organics [6] . Plants and their associated microorganisms can modify the chemistry of the soil in contact with roots, leading to rock weathering [29] , [30] , [31] . Such weathering effects take place through changes in soil pH derived from organic acids released by microorganisms [30] , and may increase the availability of inorganic compounds to plants [31] , [32] . Endolythic microorganisms can grow in gypsum by dissolving rocks, including lichens, free-living algae, fungal hyphae, cyanobacteria and non photosynthetic bacteria [24] . Furthermore, some gypsum plants like H. squamatum also show the ability to dissolve gypsum, being able to grow their roots into Petrogypsic soil horizons ( Supplementary Fig. 3 ). This ability may be related to the activity of associated root microorganisms of this species, which include arbuscular and ectomycorrhizae [33] . The ability of plants and their associate microorganisms to dissolve gypsum would also explain the use of crystallization water during spring, when gypsum is thermodynamically stable. Although the underlying mechanisms require further research, our results provide the first evidence in support of the role of gypsum crystallization water as a water source for life. These results significantly modify the current paradigm on water use by plants, where water held in the crystalline structure of mineral rocks is not regarded as a potential source. Given the demonstrated existence of gypsum on the surface of Mars [5] and its widespread occurrence on arid and semi-arid regions worldwide [2] , [3] , [4] , our results have important implications for exobiology, the study of life under extreme conditions and arid land reclamation and use. Study site and species Field records were taken in the nearly-pure gypsum outcrops between Villamayor and Alfajarín, 2–8 km East of Zaragoza, Middle Ebro Valley, Northeastern Spain (41°37′49′′N 0°41′18′′W, at 320 m above sea level). The dominant substratum in this area is gypsum, with a few thin inserted outcrops of marls and clays [34] . Almost-pure flour-like gypsum soils (with gypsum contents typically >60–70%), such as the ones included in this study, are particularly stressful areas due to their low water retention and fertility [12] . Climate is semi-arid and highly seasonal, with a mean annual temperature of 14.6 °C, and an average annual rainfall of 326 mm, which falls mainly during spring and autumn [35] ( Supplementary Fig. 4 ). The species selected for study was H. squamatum (L.) Pers (Cistaceae), a small (10–30 cm), evergreen, woody sub-shrub that is mainly distributed in the eastern half of the Iberian Peninsula, with additional localities in Northern Algeria [36] . It grows exclusively on gypsum soils and is considered a diagnostic species of Iberian gypsum vegetation [37] , [38] . It shows a delayed phenological pattern, with shoot growth taking place between March and May and flowering from May to August [13] . Its root system is shallow, with a maximum root depth of 65 cm and most fine roots occurring in the top 25 cm of the soil [11] . To explore the generality of our results, we analyzed another three shallow-rooted species that coexist with H. squamatum in the study area. These included: the gypsum-specialist Lepidium subulatum L., and the non-specialists: Linum suffruticosum L. and Helianthemum syriacum (Jacq.) Dum. Cours. All of them are small woody sub-shrubs with a similar architecture to H. squamatum and shallow root systems [11] . Due to their shallow roots and their preferred distribution on the slope of gypsum hills, these species do not have access to the water table [12] . Consequently, rain or dew water stored as free water in the soil and the crystallization water of gypsum are the only potential sources of water for them. Plant and soil sampling for isotope analyses Field sampling for isotope analyses was undertaken in spring (24 May) and summer (28 August) 2012. On each sampling date, the main stems (including the upper coarse root portion) of five individuals of study species were harvested. Vigorous, medium-sized individuals located at least 5 m away from each other were selected for sampling. To maximize the representativeness of xylem water as an indicator of the water sources used by plants and to minimize the risk of stem water evaporation, harvest was performed during mid-morning (7–9 h solar time), when maximum transpiration rates are expected in dry environments [39] , and evaporative demand is low [20] . The bark and phloem were scraped off the stems with a knife to avoid the evaporative surface of the stem and contamination with organic compounds present in living cells and/or the bark [16] . Soil samples were collected from soil in direct contact with excavated plant roots at two different depths: 0–10 cm and 10–20 cm. All individual plants collected had most of their fine roots within the upper 20 cm of the soil, following the standard distribution pattern of their respective species. Right after harvest, stem and soil samples were placed in individual airtight sealed cultivar tubes (Duran GL18), immediately frozen in the field with dry ice, and kept frozen until distillation. Water extraction Xylem and soil water were extracted by cryogenic vacuum distillation [16] at the Laboratory of Silvicuture of the Universitat de Lleida. Sample tubes were placed in a heated silicone oil bath, and connected with Ultra-Torr unions (Swagelok Company, Solon, OH, USA) to a vacuum system ( ca . 10 −2 mbar) including U-shaped water traps in series that were cooled with liquid N 2 . After an extraction time of 2 h, captured water was transferred into cap-crimp 2 ml vials, and stored at 4 °C until analysis. According to previous tests, 40–90 min are needed to obtain a complete distillation of xylem water and free water in clay soils, but shorter times are enough for sandy-lime soil samples [40] , [41] . The temperature of the bath varied depending on the type of water to be extracted. Xylem water was directly distilled at 120 °C, whereas a stepwise distillation was performed in gypsum soils, first at 35 °C, then at 120 °C. Preliminary tests with a subset of soil samples of different origin showed that an intermediate temperature (50 °C) was able to extract some of the crystallization water, but showed inconsistent values, suggesting incomplete distillation with free water ( Supplementary Fig. 5 ). This was tested in both natural and labelled soil samples. As natural samples, we used soils from the pots used in the drought experiment (collected together with the plants in May 2013, see details below), sampled just after the experiment or after drying for 3 weeks at ambient conditions, plus two additional soil samples collected in the study area in March and April 2013. The ability of the method to separate free and crystallization water was also evaluated with samples in which crystallization water was labelled with water with a known isotopic composition ( Supplementary Fig. 5b ). To obtain these modified gypsum soil samples we dehydrated natural gypsum soil at 120 °C for 3 days, to convert gypsum to bassanite and anhydrite through dehydration. We then rehydrated bassanite to gypsum by incubating for 3 days in water of known isotopic composition, including: snow water ( δ 18 O=−15.00‰, δ 2 H=−53.94‰), boiled water ( δ 18 O=+0.23‰, δ 2 H=−29.12‰), and D 2 O-labelled water ( δ 18 O=−11.57‰, δ 2 H=+468.79‰) obtained by preparing a 1:10,000 dilution of D 2 O (99% atom, Sigma-Aldrich) with tap water. After rehydration, snow- and boiled-labelled samples were left drying at ambient conditions for 3 days and then sampled in sealed glass tubes as described above, whereas D 2 O-labelled samples were left drying for 3 weeks prior to sampling. The original isotopic composition of the mother water was calculated from measured crystallization water by applying fractionation factors for the incorporation of water into gypsum ( α 18 O=1.004 (ref. 42 ), and α 2 H=0.98, (ref. 43 )): In all tested samples, we found large variations in free water, in agreement with the expected fractionation effects of soil drying [15] ( Supplementary Fig. 5 ): values within the meteoric water line in soils at field capacity (control), enrichment in moderately dry samples (control-dried, drought, and snow- and boiled-labelled), and depletion in very dry samples (drought-dried, D 2 O-labelled). Natural samples showed rather constant values for crystallization water ( Supplementary Fig. 5a ), while in labelled samples crystallization water varied according to the isotopic composition of labelling water ( Supplementary Fig. 5b ). The amount of free soil water extracted after distillation at 35 °C varied significantly between sampling dates ( F =14.4, P =0.004), indicating a decrease in soil moisture during summer. The decrease was more significant in the bottom soil (spring=2.0±1.07%, summer=0.6±0.07% dry soil weight; F =8.4, P =0.04) than in the top soil (spring=1.3±0.06%, summer=0.5±0.17% dry soil weight; F =5.3, P =0.08). No significant change was detected between sampling dates or soil depths in the amount of crystallization water extracted ( F =1.0, P =0.326). For the soil samples in the pot experiment, we also compared the amount of water recovered at 35 °C with the soil water content (SWC) determined gravimetrically in the pots (see details in section ‘drought experiment’). The tight relationship obtained further supports a complete recovery of free water from the soil after distillation ( SWC gravimetric =0.8412 × SWC distillation +0.0116, r 2 =0.966, N =10). Stable isotope analyses δ 2 H and δ 18 O analyses were determined by cavity ring-down spectroscopy (CRDS) at the Serveis Científico-Tècnics of the University of Lleida (Lleida, Spain), using a Picarro L2120-i, coupled to a high-precision vaporizer A0211. For each sample, six replicates of 1 μl were injected into the vaporizer, keeping the last three injections for calculation. Overall uncertainty (determined as the standard error of repeated analyses ( N =20) of a reference sample not included in the calibration) was 0.05 and 0.17‰, for δ 18 O and δ 2 H, respectively. In autumn 2012, the system was upgraded with a Micro-Combustion Module (MCM), which is located between the vaporizer and the CRDS. Once the sample is evaporated, all the gaseous phase is forced to pass through a carrier gas in which oxidation process converts the organics into minute quantities of carbon dioxide and nascent water. All samples from spring were analyzed without the module, while the samples from summer were analyzed with the new system. Several studies have shown that organic contaminants may interfere with water isotope analyses using CRDS [44] . The presence of contaminants was assessed with the Picarro software Chemcorrect 1.2.0, which assigns metrics describing the magnitude of contamination as well as the potential source, and includes flagging indicating contamination degree by a colour code: green for not contaminated samples, yellow for possibly contaminated samples and red for very contaminated samples. When analyzed without the MCM module ( N =41), 63.4%, 12.2% and 24.4% of the samples were labelled as green, yellow and red, respectively. Using the MCM module ( N =124), 87.1%, 6.5% and 6.5% of the samples were labelled as green, yellow and red, respectively. It should be noted that, with the MCM, only Lepidium samples showed a true contamination. Other flagged samples were soil samples extracted at 50 °C, which showed high standard deviation due to insufficient amount of sample in the last injections, and deuterated samples, due to their unusual spectral features. Although corrected values are not directly provided, Chemcorrect also incorporates corrected peaks for H 2 18 O, HD 16 O and H 2 16 O, which can be directly converted into raw isotope values by applying factory calibration values, which are available for each Picarro unit. To check the reliability of the MCM and post-processing corrections, a subsample of water extracts from six soil and six xylem samples, selected to cover the observed range of organic contamination, was used to compare the different methods: with or without the MCM module and with or without applying the software correction ( Supplementary Fig. 6 ). As reference values, the samples were analyzed by Isotope Ratio Mass Spectrometry at the laboratory of atmospheric chemistry (Paul-Scherrer-Institute, Villigen, Switzerland). An aliquot of 0.6 μl of the water sample was injected in a High Temperature Combustion Elemental Analyzer (TC/EA, Thermo Finnigan, Bremen, Germany). At 1,450 °C, the water was pyrolyzed on glassy carbon to H 2 and CO, and then these components were carried in a helium stream to the mass spectrometer (Delta plus XP, Thermo Finnigan). The hydrogen isotope ratio was determined from the 2 H/ 1 H ratio of the H 2 molecule and the oxygen isotope ratio from the 12 C 18 O/ 12 C 16 O ratio of the CO molecule. The values are expressed as deviations in ‰ from the international standard Vienna Standard Mean Ocean Water (VSMOW, δ 18 O, δ 2 H). The overall uncertainty for the measurements was <0.2‰ for δ 18 O and <1.0‰ for δ 2 H. The Local Meteoric Water line was calculated from monthly isotope data from Zaragoza for the period 2000–2006, made publicly available by the Global Network of Isotopes in Precipitation [45] . Drought experiment On 24 May 2013, 20 H. squamatum plants were lifted from the field (41°41′50′′N, 0°44′42′′W) and planted in 0.006 m −3 pots. Plants were left to stabilize for 2 months in a shaded tunnel, with regular tap watering to keep soil moist. On 16 August 2013, half of the plants were allocated to the control treatment (daily watering to field capacity) and the other half to the drought treatment (no watering). The soil water content of pots was evaluated gravimetrically every afternoon just before watering, and referred to the dry weight of pots, determined after drying at ambient temperature for 3 weeks. Volumetric water content at field capacity was estimated based on the water content of control pots after watering and allowing to drain for 1 h. Gas exchange measurements were taken with an Infrared Gas Analyzer (Walz GFS3000, Heinz Walz GmbH, Effeltrich, Germany) at early and late morning, 4 and 7 days after the beginning of the application of treatments. At each time, measurements were taken in one twig per plant, inserted in a standard measuring head (chamber volume: 6 cm 3 ) equipped with a light source (LED-Array/PAM Fluorometer 3055-FL). Ambient CO 2 was fixed to 400 p.p.m., and flow rate to 750 mol s −1 . Temperature, relative humidity and Photosynthetic Photon Flux Density in the chamber were set to 20 °C, 65%, 500 μmol m −2 s −1 in the early morning, and 32 °C, 50%, 1,200 μmol m −2 s −1 in the late morning, emulating outside conditions. All parameters were recalculated to actual leaf area using the equations from von Caemmerer and Farquhar [46] . Leaf area was determined by taking a digital image, measuring the mean area of the leaves that were located horizontally in the chamber (Image J 1.42q, Wayne Rasband, the National Institute of Health, USA), and multiplying it by the total number of leaves inside the chamber. Leaf area per plant was determined by measuring projected area with Image J, and correcting for the observed relationship between projected area and actual area (actual=1.4869 × projected+0.4568, R 2 =0.6144, N =47, P <0.001). With these values, transpiration rates per leaf area were extrapolated to the whole plant. On 23 August 2013, plants were harvested and the fresh and dry weight (48 h at 60 °C) of the stems was measured to estimate total water content in above ground xylem. The mean xylem water residence time was subsequently calculated as the ratio between the total water content in the xylem and the extrapolated total transpiration per plant. Calculations and statistical analyses Differences in the isotopic composition of the xylem sap of H. squamatum plants between seasons were evaluated by general linear models (GLM) with ‘season’ as fixed factor. Differences in the isotopic composition of the xylem sap of H. squamatum and that of coexisting shallow-rooted species were analyzed by GLM models with ‘species’ and ‘season’ as fixed factors. Differences between seasons and sources of water in the isotopic composition of soil water in the field, and between sampling dates, time of the day and treatments in gas exchange parameters in the pot experiment, were analyzed by residual maximum likelihood (REML) models with ‘season’ and ‘sources’ or ‘date’, ‘time of the day’ and ‘treatment’, respectively, as fixed factors. Similarly, differences in the amount of free and crystallization water extracted by cryogenic distillation between sampling dates and soil depths were analyzed by REML models with ‘season’ and ‘depth’ as fixed factors. To analyze differences in the amount of free and crystallization water extracted from each sampling depth, REML models were also run with ‘season’ as a fixed factor separately for each soil depth. All REML models included ‘plant ID’ as a random factor to account for spatial autocorrelation between soil samples collected underneath the same plant, in the case of isotopic and soil water content data, and the repeated measures effects, in the case of data from the drought experiment. When significant, differences between groups were evaluated by post-hoc honestly significant difference-Tukey tests. All data were normally distributed (as assessed by normal quantile plots with Lilliefors 95% confidence limits) except for water residence time that was log-transformed to meet normality. Homogeneity of variances was checked visually by plotting residuals against factors [47] and applying Levene’s test for homogeneity of variances when in doubt. Heterogeneous data were analyzed by including the varIdent structure in GLM and REML models (the nmle package [47] ). This structure allows for different variances among the different strata of the categorical factors included in models [47] . The relative contribution of different water sources to the composition of the xylem sap was estimated using the package SIAR for R, which solves mixing models for stable isotopic data based upon a Gaussian likelihood with a dirichlet prior mixture on the mean [48] . The model uses as input, multiple isotope values of ‘consumers’ (in our case individual values of δ 18 O and δ 2 H for each plant), sources (mean plus standard deviation) and a correction matrix for potential fractionation (set to 0 for both isotope pairs). We set the number of iterations to 500,000, the size of burnin to 50,000, and the amount of thinning for the final output to 10,000 iterations. For calculations we used two different functions. First, we used the standard ‘siarmcmcdirichletv4’, in which the output is calculated on a population-basis, classifying individual plants into different groups (in our case, spring and summer). The command does not allow having separate source matrices for each group, and requires at least two groups. Thus, we run the model for the two groups of plants, including either spring or summer sources, but considered only the output data for the relevant group (spring or summer). This is the most recommended method, since it considers population variability when estimating source proportions. Alternatively, we also run the ‘siarsolomcmcv4’ function to obtain separate estimates for each of the plants. The input data is the same, but in this case calculations were done separately for each plant, including five plants in each run (spring and summer). All statistical analyses were run in R 2.14.1 (R Core Team, 2012). How to cite this article: Palacio, S. et al . The crystallization water of gypsum rocks is a relevant water source for plants. Nat. Commun. 5:4660 doi: 10.1038/ncomms5660 (2014).